Enhancing lithium–sulphur battery performance by strongly binding the discharge products on amino-functionalized reduced graphene oxide Lithium–sulphur batteries are one very appealing power source with high energy density. But their practical use is still hindered by several issues including short lifespan, low efficiency and safety concern from the lithium anode. Polysulphide dissolution and insulating nature of sulphur are generally considered responsible for the capacity degradation. However, the detachment of discharge products, that is, highly polar lithium sulphides, from nonpolar carbon matrix (for example, graphene) has been rarely studied as one critical factor. Here we report the strongly covalent stabilization of sulphur and its discharge products on amino-functionalized reduced graphene oxide that enables stable capacity retention of 80% for 350 cycles with high capacities and excellent high-rate response up to 4 C. The present study demonstrates a feasible and effective strategy to solve the long-term cycling difficulty for lithium–sulphur batteries and also helps to understand the capacity decay mechanism involved. Advanced power source is urgently needed to meet the continuously surging demand in consumer electronics and electric vehicles. Although lithium (Li)-ion batteries have been successful in powering portable electronics, they face many challenges such as safety, cost and energy density for large-scale applications, for example, as the power supply to drive electric vehicles for 300–500 miles per charge. This boosts a great deal of interest in seeking for high-performance batteries that can store and deliver more electric energy efficiently. Lithium–sulphur (Li–S) batteries are one of the prospective candidates in this regard because of the inherently high theoretical energy density of 2,567 Wh kg −1 given by the redox reaction between elemental sulphur and Li (normally expressed as S 8 +16Li↔8Li 2 S) [1] , [2] , [3] , [4] . This value is almost one order of magnitude higher than that of popular Li-ion batteries based on intercalation compound (for example, LiCoO 2 and LiFePO 4 ) cathodes. Features such as low cost (~$150 per ton), non-toxicity and natural abundance of sulphur also bring extra benefit to the market potential [5] . Typically, a rechargeable Li–S cell consists of a sulphur cathode and Li anode, with an organic liquid electrolyte as both the charge-transfer medium and the ionic conductor. It operates by the successive reduction of sulphur to various soluble polysulphides (Li 2 S x , x >2) and insoluble lithium sulphides (Li 2 S x , 1≤ x ≤2) at the cathode upon discharge and reverse reaction upon charge [6] . Complex sulphur chemistries generate the high energy density, but at the same time predetermine several critical difficulties for commercialization of Li–S batteries: (i) the insulating nature of sulphur (5 × 10 −30 S cm −1 ) causes very low utilization of the active material; (ii) the high solubility of polysulphide intermediates in organic liquid electrolyte leads to the active mass loss and the notorious shuttle effect; and (iii) the marked volume change of sulphur (~80%) upon lithiation/delithiation reduces the mechanical integrity of the electrode. Using sulphur–carbon composites has been regarded as a major approach to enhance the conductivity and stability of sulphur cathodes [1] , [5] , [7] , [8] , [9] , [10] , [11] , [12] , [13] , [14] , [15] , [16] , [17] , [18] , [19] , [20] , [21] , [22] , [23] , [24] , [25] , [26] , [27] . However, the physical barriers provided by sequestration and adsorption in carbon materials can only slow down the sulphur loss in a short term owing to the weak interactions between nonpolar carbon and highly polar polysulphides [1] , [7] , [8] , [9] , [10] , [11] , [12] , [13] , [14] , [15] , [16] , [17] , [18] , [19] , [20] , [21] , [22] . Indeed, migration of ionic polysulphide species is hard to be completely prevented by physical adsorption in carbon since it is driven by electrical field in the electrolyte. Hence strong chemical binding of sulphur and its discharge products to the carbon host is fundamentally essential to eliminate the polysulphide shuttling. On the other hand, protection of the metallic Li anode against redox side reactions in flammable liquid electrolyte might be another strategy to alleviate the polysulphide shuttling and safety hazards (for example, short circuits and fires) caused by dendritic growth of Li [6] . To this end, various additives such as LiNO 3 and P 2 S 5 have been used to passivate the Li anode in organic electrolyte, achieving high Coulombic efficiency of over 90% (refs 6 , 28 ). However, gradual consumption of additives on the electrodes leads to a decrease in the protection efficiency. Replacing flammable liquid electrolytes with high-conductivity solid electrolytes brings some interesting perspective to address the polysulphide dissolution related issues in Li–S cells [29] , [30] . Nevertheless, development of all solid-state Li–S batteries is still largely limited owing to lack of solid electrolytes with conductivity comparable to that of liquid electrolytes. Polysulphide dissolution represents a common, but not the sole reason for the capacity decay of sulphur cathodes. Investigations by in operando transmission X-ray microscopy and inductively coupled plasma-optical emission spectroscopy have revealed that dissolution of sulphur in electrolyte is not so severe and just takes limited responsibility for the capacity fading [31] , [32] . Recently, the detachment and separation of lithium sulphides (Li 2 S x , 1≤ x ≤2), the full-discharge products, from the carbon matrix was identified as another important, but rarely noticed, contributing factor to cause irreversible active mass loss and electrical contact isolation. To mitigate this problem, amphiphilic polymers such as polyvinylpyrrolidone are introduced to modify the interfacial properties of sulphur–carbon composites, achieving a long lifespan of 300 cycles at 0.5 C (ref. 27 ). Nevertheless, the rate capability of cells is still limited by non-covalent adsorption of the poorly conductive polymer shell on carbon surface. Herein, we report a facile approach towards high-performance sulphur-carbon cathodes by covalently stabilizing the sulphur and its discharge products on amino-functionalized reduced graphene oxide (rGO). Specifically, ethylenediamine (EDA) is chosen to demonstrate our concept because it is a Lewis base composed of two electron-donating amine groups on a carbon aliphatic (CH 2 –CH 2 ) spacer. This unique molecular structure with high reactivity makes it an ideal crosslinker to covalently join polar lithium sulphides and nonpolar carbon surface together, which effectively prevents loss of active mass and electrical contact. The strong affinity of lithium sulphides to EDA-functionalized rGO (EFG) is verified by density-functional theory (DFT) calculation, as characterized by high binding energy of 1.13–1.38 eV between them. In addition, the electron-donating effect of EDA moieties also enhances the reactivity of aromatic carbon rings for sulphur loading and favours the immobilization of sulphur by complexation with it. With the merits of rGO such as good conductivity and flexible structure, the nanocomposite of EDA-functionalized rGO and sulphur (denoted as EFG–S) exhibits exceptionally stable capacity retention of 80% for 350 cycles with high capacities and excellent high-rate response up to 4 C for 200 cycles. Synthesis and characterizations of the EFG–S nanocomposite Two facile steps are involved to synthesize the EFG–S nanocomposite. First, EDA moieties are grafted onto GO by nucleophilic attack to the epoxy carbon and β-carbon of –OH groups on GO surface at 75 °C (ref. 33 ). This process simultaneously reduces electrically insulating GO to conductive rGO (170 S cm −1 ) with the removal of oxygen-containing groups. The inter-linkage of rGO sheets is inhibited by precise control over the precursor concentration and reaction temperature that facilitates the subsequent sulphur loading. Next, sulphur is loaded to EFG by the disproportionation reaction of Na 2 S 2 O 3 in dilute hydrochloric acid, followed by annealing at 155 °C in Ar. Scanning electron microscopy (SEM) together with transmission electron microscopy (TEM) characterization reveals that the resultant EFG–S nanocomposite consists of wrinkled nanosheets with uniform coverage of sulphur on the external surface ( Fig. 1a,b ). No large sulphur particles are observed in the sample. We fail in obtaining a high-resolution TEM image of the sulphur nanoparticles because they sublimate very fast under electron beam irradiation. However, homogenous distribution of sulphur in the nanocomposite can be verified by elemental mapping, as shown in Fig. 1c,d . Thermogravimetric analysis and elemental analysis suggest that the overall content of sulphur in the EFG–S nanocomposite is ~60–69 wt.% with 11–14 wt.% of EDA moieties ( Supplementary Fig. 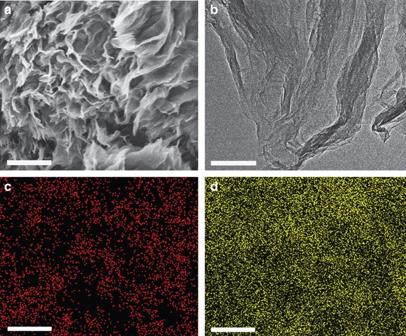Figure 1: Characterizations of EFG–S nanocomposite. (a) SEM (scale bar, 500 nm) and (b) TEM images (scale bar, 100 nm) of EFG–S nanocomposite. (c,d) Elemental mapping showing the homogenous distribution of carbon and sulfur on EDA-functionalized rGO, respectively (scale bars, 500 nm). 1 and Supplementary Table 1 ). Figure 1: Characterizations of EFG–S nanocomposite. ( a ) SEM (scale bar, 500 nm) and ( b ) TEM images (scale bar, 100 nm) of EFG–S nanocomposite. ( c , d ) Elemental mapping showing the homogenous distribution of carbon and sulfur on EDA-functionalized rGO, respectively (scale bars, 500 nm). Full size image The structural characteristics of the EFG–S nanocomposite are determined by powder X-ray diffraction (XRD), as shown in Supplementary Fig. 2a . All the pronounced peaks can be assigned to orthorhombic sulphur (JCPDS card no. 08-0427) with high crystallinity. For both EFG and EFG–S samples, no diffraction peaks from GO appear owing to the effective reduction of GO, and the absence of rGO restacking is also verified. The removal of oxygen-containing groups by EDA functionalization is further evidenced by Fourier transform-infrared spectroscopy (FTIR), as shown in Supplementary Fig. 2b . In the spectrum of GO, the absorption peaks at 1,720, 1,390, 1,224 and 1,059 cm −1 can be ascribed to stretching vibrations of C=O, –OH, carbonyl C–O and epoxy C–O bonds, respectively [16] . The absorption peaks at 3,000–3,600 cm −1 correspond to the O–H stretching vibrations of hydroxyl groups on GO surface and adsorbed water molecules. After reacting with EDA, the intensity of these peaks is greatly suppressed, while new peaks arise at 1,564, 1,150–1,465 and 3,430 cm −1 that can be assigned to the antisymmetric C–N stretching vibrations coupled with out-of-plane NH 2 and NH modes, as well as the N–H stretching vibrations [22] , [34] , [35] . The scissoring in-plane bending mode of primary –NH 2 groups is also observed at 1,633 cm −1 by overlapping with the peaks from C–C aromatic ring modes at 1,615 cm −1 (ref. 36 ). Overall, the above results clearly indicate the strong covalent linkage of EDA moieties to rGO. After sulphur loading, however, most of the peaks disappear in the FTIR spectrum owing to the infrared inactivity of the sulphur layer. Thus X-ray photoelectron spectroscopy (XPS) is used to detect the variation of elemental composition and functional groups in the samples, as shown in Fig. 2 . In the C 1 s spectra, the intensity of the peak corresponding to sp 2 -hydridized carbon (at 284.6 eV) increases continually from GO to EFG and EFG–S, while the change of oxygen signals (286.5 eV for C–O, 287.4 eV for C=O and 288.9 eV for O–C=O groups) shows the opposite trend [8] . This observation is consistent with the above XRD and FTIR results, revealing the effective removal of oxygen-containing groups from GO and partial restoration of the conjugated graphene sheets. In Fig. 2b,c , the presence of amine groups in the EFG and EFG–S samples is confirmed by the peak at 285.6–285.8 eV for the C–N bond in the primary amine [36] . The peak at 285.6 eV in XPS C 1 s spectrum of the EFG–S sample is partially ascribed to the C–S bonds, revealing the chemical bonding between elemental sulphur and rGO. The successful loading of sulphur on EFG is also depicted by the S 2 p spectrum of EFG–S, as characterized by the S 2 p 3/2 and 2 p 1/2 doublet with an energy separation of 1.2 eV and intensity ratio of ~2:1 (ref. 23 ). The binding energy of S 2 p 3/2 peak is 163.8 eV, which is slightly lower than that of elemental sulphur (164.0 eV), revealing the possible presence of C–S species [23] , [37] . The minor peaks at 168.2–168.8 eV are due to the sulphate species formed by sulphur oxidation in air [8] . In addition, the N 1s spectra of EFG and EFG–S samples show the domination of pyrrolic-type N peak at 399.5–399.8 eV, which further confirms the chemical bonding between rGO and EDA moiety before and after sulphur loading ( Supplementary Fig. 3 ) [33] . 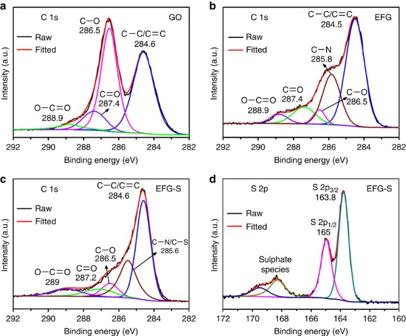Figure 2: XPS analysis of GO, EFG and EFG–S. C 1sXPS spectra of (a) GO, (b) EFG and (c) EFG–S nanocomposite. (d) S 2pXPS spectrum of EFG–S nanocomposite. Figure 2: XPS analysis of GO, EFG and EFG–S. C 1 s XPS spectra of ( a ) GO, ( b ) EFG and ( c ) EFG–S nanocomposite. ( d ) S 2 p XPS spectrum of EFG–S nanocomposite. Full size image Electrochemical performance The electrochemical Li storage in the EFG–S nanocomposite is studied by cyclic voltammetry (CV) analysis within a cutoff voltage window of 1.5–3.0 V at a scan rate of 0.1 mV s −1 , as shown in Supplementary Fig. 4 . During the first cycle, two pronounced peaks are observed on the cathodic curve at ca. 2.35 and 2.04 V owing to the multistep reduction of elemental sulphur with Li. Specifically, the peak at ~2.35 V can be ascribed to a solid-to-liquid (from S 8 to dissolved Li 2 S 8 ) phase transition while the one at ~2.04 V is associated with a liquid-to-solid phase transition from dissolved lithium polysulphides to lithium sulphides [6] . The anodic peak at ~2.35 V is owing to the formation of Li polysulphides (Li 2 S x , 2< x ≤6), which proceeds until the S 8 ring is restored at 2.4 V (refs 13 , 38 ). The CV curves at subsequent cycles show good reproducibility with complete overlapping of all the peaks, suggesting a very high degree of reversibility of the multistep reactions. When evaluated as a cathode material for Li–S batteries, the EFG–S nanocomposite exhibits excellent electrochemical performance. 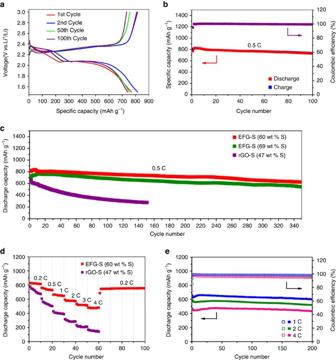Figure 3: Electrochemical measurements. (a) Discharge/charge voltage profiles of EFG–S nanocomposite for the 1st, 2nd, 50th and 100th cycles; (b) cycling performance and Coulombic efficiency of EFG–S nanocomposite; (c) long-term cyclability of EFG–S nanocomposite (60 and 69 wt.% S) and rGO–S composite (47 wt.% S). All these tests are conducted at 0.5 C between 1.5 and 3.0 V. (d) Rate capabilities of EFG–S and rGO–S nanocomposites, which are obtained between 1.5 and 3.0 V at various current densities. (e) Cycling performance and Coulombic efficiency of EFG–S nanocomposite (60 wt.%) at 1, 2 and 4 C. Figure 3a shows representative discharge/charge voltage profiles of the EFG–S nanocomposite at a current rate of 0.5 C (1 C=1,672 mA g −1 ) in the voltage window of 1.5–3.0 V. Consistent with reports in literature and above CV analysis, typical two-plateau behaviour is observed, corresponding to the formation of long-chain (high plateau at 2.35 V) and low-order (low flat plateau at 2.0 V) polysulphides during discharge [5] , [8] . Instead of rapid initial decay in capacity generally reported for sulphur cathodes [5] , [7] , [12] , [15] , the discharge capacity gradually increases from 770 mAh g −1 for the first cycle to 820 mAh g −1 after several cycles, indicating strong affinity of the discharge products on functionalized rGO. Such a capacity rise was also observed for the nanocomposite of sulphur and hollow carbon nanofibres modified with amphiphilic polymers [27] . It should be noted that rGO in the EFG–S nanocomposite is electrochemically inactive in the voltage window tested, therefore, it does not contribute to the observed capacity. From the second cycle onwards, the EFG–S nanocomposite exhibits stable capacity retention of over 90% for 100 cycles with high Coulombic efficiency of nearly 100%, as shown in Fig. 3b , thereby suggesting little polysulphide shuttling. After deep cycling for as many as 350 cycles, a high capacity of 650 mAh g −1 can still be retained corresponding to a high capacity retention of ca. 80% ( Fig. 3c ). The observed superior cyclability is also repeatable for the EFG–S nanocomposite with a higher sulphur loading of 69 wt.% that exhibits stable capacity retention of 75% over 350 cycles at the same current rate ( Fig. 3c ). To fully demonstrate the advantages of EFG–S nanocomposites, cycling performance of the rGO-sulphur (rGO–S, 47 wt.% S) nanocomposite is also investigated under the same conditions. In a vast contrast, the rGO–S nanocomposite exhibits lower capacity with fast capacity decay in 150 cycles. Figure 3: Electrochemical measurements. ( a ) Discharge/charge voltage profiles of EFG–S nanocomposite for the 1st, 2nd, 50th and 100th cycles; ( b ) cycling performance and Coulombic efficiency of EFG–S nanocomposite; ( c ) long-term cyclability of EFG–S nanocomposite (60 and 69 wt.% S) and rGO–S composite (47 wt.% S). All these tests are conducted at 0.5 C between 1.5 and 3.0 V. ( d ) Rate capabilities of EFG–S and rGO–S nanocomposites, which are obtained between 1.5 and 3.0 V at various current densities. ( e ) Cycling performance and Coulombic efficiency of EFG–S nanocomposite (60 wt.%) at 1, 2 and 4 C. Full size image In addition, the EFG–S nanocomposite also shows excellent cycling response to continuously varying current densities despite that sulphur cathodes are generally observed to suffer from sluggish kinetics and poor conductivity ( Fig. 3d and Supplementary Fig. 5 ). While cycled at high rates of 1–4 C, comparable capacities of ca. 480–660 mAh g −1 can be still retained. After deep cycling at 4 C, stable high capacity could be largely restored for repeated cycles after abruptly switching the current rate back to 0.2 C, indicating the excellent robustness and stability of the nanocomposite. As a comparison, the rate performance of the rGO–S nanocomposite is also shown in Fig. 3d , which is expectedly inferior to that of the EFG–S nanocomposite. The long-term cycling tests show that the EFG–S nanocomposite could exhibit high capacity retention of over 90% for 200 cycles at high rates of 1–4 C ( Fig. 3e ). Such remarkable high-rate performance is superior to that of rGO–S composite and most reported carbon–sulphur nanocomposites, which lose almost all of the capacity upon cycling under similar high rates [5] , [7] , [8] , [12] , [13] , [14] , [16] , [18] , [27] . Apparently, the EDA functionalization has a critical role for enhancing the lifespan and rate capability of EFG–S nanocomposites. Interaction between lithium sulphides and EFG When the electroactive materials are reduced upon full discharge, strong affinity of lithium sulphides (Li 2 S x , 1≤ x ≤2) to the carbon matrix is reasonably vital to retain the active mass and electrical contact of the composite. SEM and TEM images of the EFG–S electrode in the discharged state after 350 cycles reveal that the discharge products are uniformly coated on EFG surface to form a thick layer instead of discrete particles, implying the strong interaction between them ( Fig. 4a,b ). The homogeneous distribution of lithium sulphides on graphene sheets is confirmed by elemental mapping ( Fig. 4c,d ). For the discharged rGO–S nanocomposite after 150 cycles, however, nanosheet structures with relatively bare surface are observed as a result of significant detachment of the discharge products from carbon surface ( Fig. 4e–h ). To further understand the interaction between the discharge products and the carbon surface, DFT calculations are performed by taking Li 2 S and single-layer graphene as the model system. The results suggest that the binding energy between Li 2 S clusters and pristine graphene (0.34 eV; Fig. 4i ) is much lower than that of sulphur and graphene (0.79 eV) [27] . The weakened adhesion of lithium sulphides to carbon surface inevitably causes the detachment and separation of electroactive materials from the carbon matrix, which coupled with polysulphide dissolution, leading to inferior performance of most sulphur-carbon composites. After EDA functionalization, Li 2 S can bind to EDA moieties in two ways: to nitrogen atom of the amine group with smallest steric hindrance ( Fig. 4j ) or to both nitrogen atoms of EDA moiety for stronger binding ( Fig. 4k ), corresponding to high binding energies of 1.13 and 1.38 eV, respectively. On the other hand, DFT calculation also confirms the strong chemical bonding between the EDA moieties and rGO. In EFG, the EDA moieties are grafted on rGO surface by covalent C–N bonds with a high binding energy of 2.58 eV and bond length of 1.5 Å, which is consistent with FTIR and XPS analyses. After full discharge, high binding energies of 2.08–2.30 eV can still remain for strongly binding the EDA moieties to rGO ( Fig. 4j,k ). As a result, the detachment and separation of lithium sulphides from the carbon matrix could be effectively suppressed to achieve superior electrode stability for long-term charge/discharge cycling. To further investigate the interaction between EDA moieties and lithium sulphides, XPS analysis was performed for the EFG–S electrode after full discharge to 1.5 V ( Supplementary Fig. 6 ). The Li 1 s spectrum can be fitted with two peaks at 54.6 and 55.4 eV, which can be attributed to Li–N and Li–S bonds, respectively [38] , [39] . The binding energy of N 1 s peak is slightly reduced to 399.2 eV perhaps owing to the interaction with the less electronegative atom such as Li. In the S 2 p spectrum after discharge, the dominant peak at 161.5–162.7 eV can be ascribed to Li–S bonds in lithium sulphides while signals from elemental sulphur disappear completely [38] . The appearance of Li–N peaks, alongside the shift of N 1 s peak, clearly indicates the strong interaction between the EDA moieties and discharge products. This result is in good agreement with the DFT calculation results. 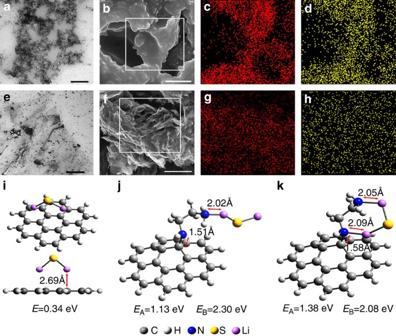Figure 4: Postmortem studies and theoretical calculations. (a) TEM (scale bar, 100 nm) and (b) SEM image (scale bar, 5 μm) of EFG–S nanocomposite in the discharged state after 350 cycles. (c,d) Elemental mapping showing the homogenous distribution of carbon and sulfur in the composite, respectively. (e) TEM (scale bar, 100 nm) and (f) SEM image (scale bar, 1 μm) of rGO–S nanocomposite in the discharged state after 150 cycles. (g,h) Elemental mapping showing the presence of carbon and sulfur in the composite, respectively. The cells were discharged to 1.5 V before the characterization. DFT calculation showing the interaction between Li2S cluster and (i) single-layer graphene or (j,k) EFG.EAis defined as the binding energy between Li2S and EFG.EBis defined as the binding energy between EDA–Li2S and graphene. All the models are shown in the most stable configuration. In the models, the carbon (C), hydrogen (H), nitrogen (N), sulphur (S) and lithium (Li) elements are displayed as spheres in grey, white, blue, yellow and pink, respectively. Figure 4: Postmortem studies and theoretical calculations. ( a ) TEM (scale bar, 100 nm) and ( b ) SEM image (scale bar, 5 μm) of EFG–S nanocomposite in the discharged state after 350 cycles. ( c , d ) Elemental mapping showing the homogenous distribution of carbon and sulfur in the composite, respectively. ( e ) TEM (scale bar, 100 nm) and ( f ) SEM image (scale bar, 1 μm) of rGO–S nanocomposite in the discharged state after 150 cycles. ( g , h ) Elemental mapping showing the presence of carbon and sulfur in the composite, respectively. The cells were discharged to 1.5 V before the characterization. DFT calculation showing the interaction between Li 2 S cluster and ( i ) single-layer graphene or ( j , k ) EFG. E A is defined as the binding energy between Li 2 S and EFG. E B is defined as the binding energy between EDA–Li 2 S and graphene. All the models are shown in the most stable configuration. In the models, the carbon (C), hydrogen (H), nitrogen (N), sulphur (S) and lithium (Li) elements are displayed as spheres in grey, white, blue, yellow and pink, respectively. Full size image Both the experimental measurement and theoretical calculation above demonstrate the strong interaction between discharged lithium sulphides and EFG. The lone-pair electrons donated by the amine groups of EDA moieties not only trigger the nucleophilic reaction with oxygen-containing groups on GO but also interact with lithium sulphides by coordination with Li atom [20] , [33] , [34] . In addition, it is found that sulphur is easily dissolved in the mixture of EDA and the electrolyte used (bistrifluoromethanesulphonylimide/1, 3-dioxolane–1, 2-dimethoxyethane) with a significant colour change to dark brown. The UV–visible spectrum of this solution shows the fingerprint peaks at 320, 410 and 620 nm, which is consistent with that of aqueous sulphur–EDA solution composed of alkylammonium polysulphides ( Supplementary Fig. 7 ) [40] , [41] . Therefore, it might be reasonable to speculate that the presence of EDA moieties may also help to anchor the sulphur species by forming alkylammonium polysulphides on rGO surface via nucleophilic reaction in organic electrolyte [42] , [43] . It should be pointed out that the electrostatic interaction between the alkylammonium cations and polysulphide anions might be also important for the efficient entrapment of polysulphides during the extended cycling. The electron-donating effect of EDA moieties is also favourable for enhancing the reactivity of aromatic carbon rings in rGO for anchoring sulphur. On the other hand, the strong affinity of sulphur and its discharge products to EFG significantly reduces the charge-transfer resistance in the EFG–S nanocomposite, as characterized by the smaller semicircle at high-frequency region in the electrochemical impedance spectroscopy spectra ( Supplementary Fig. 8 ). With high mechanical flexibility and good conductivity, the rGO network also contributes to the electrode stability and conductivity by providing a three-dimensional electronic pathway for fast charge transfer and mitigating the lithiation/delithiation-induced volume variation upon charge/discharge cycling [16] , [23] . Working together, the synergistic contribution from EDA functionalities and rGO framework leads to high utilization of sulphur, good electronic/ionic accessibility and high electrode stability, thus achieving exceptional performance. In summary, we have demonstrated the covalent stabilization of sulphur and its discharge products on EDA-functionalized rGO, and its great contribution to high reversible capacity, excellent rate capability and exceptionally long lifespan of Li–S cells. The EDA functionalization has multiple roles in enhancing electrochemical performance of the sulphur–carbon nanocomposite: (i) as the crosslinker to ensure strong adhesion of polar discharge products to nonpolar carbon surface; (ii) facilitate the sulphur immobilization on rGO by chemical interaction; and (iii) enhance the conductivity of the composite for better electron and ion kinetics by reducing electrically insulating GO to conductive rGO. In addition, the rGO framework also grants the nanocomposite with good conductivity and high mechanical stability. With all these advantages, the synthesized EFG–S nanocomposites could deliver durable performance of 350 cycles with 80% capacity retention and superior rate response up to 4 C. We thus believe that the current strategy may offer a new way to solve the long-term cycling difficulty for sulphur–carbon cathodes and shed some light on the fabrication of high-performance Li–S batteries. Further investigations need to be conducted to enhance the safety of Li–S cells, for example, by using highly conductive solid electrolytes. Deeper and broader investigations of the Li–S reaction mechanism are also essentially important and highly desirable to provide new perspectives for understanding the details of capacity fading in Li–S batteries. With rational and delicate design, truly durable and reliable high energy density Li–S batteries could be developed to meet the demand of new applications in future. Synthesis of EDA-functionalized rGO GO was prepared via a modified Hummers’ method reported elsewhere [44] . The EFG was synthesized by heating the mixture of EDA (120 μl) and GO suspension (90 ml, 1 mg ml −1 ) at 75 °C for 6 h in a sealed glass vessel. Synthesis of EFG–S nanocomposites For the synthesis of EFG–S nanocomposite, freshly prepared EFG suspension (40 ml) was dispersed in aqueous solution of Na 2 S 2 O 3 (260 ml, 19 mM) under ultrasonication for 1.5 h, followed by slowly adding dilute hydrochloric acid (40 ml, 0.18 M) under stirring. After 1 h, the product was harvested by several filtration-rinse cycles until the effluent becomes neutral, followed by complete drying at 60 °C. The obtained sample was stored at 155 °C for 12 h in Ar in a sealed container, giving rise to EFG–S nanocomposite with 60 wt.% S. For comparison, another EFG–S nanocomposite with 69 wt.% S was also prepared by the same procedure except for using 30 ml of EFG suspension for the reaction. Synthesis of rGO–S composite The rGO is produced by thermal reduction method reported elsewhere [45] . The rGO–S composite with 47 wt.% S was prepared following the same procedure as for EFG–S nanocomposite except that the EDA was not introduced. Materials characterization The morphology of the samples was characterized with field-emission SEM (FESEM, QUANTA 450) and TEM (FEI TF30). Powder XRD patterns were recorded on a Rigaku D/Max 2400 type X-ray spectrometer with Cu Kα radiation ( λ =1.5406 Å). The surface characteristics of the samples were investigated using a Nicolet-20DXB FTIR and ESCALAB MK II XPS. The weight ratio of the sulphur and EDA moieties in the composite was determined by thermogravimetric analysis (Shimadzu, DRG-60) and a vario EL III Elemental Analyzer (Elementar, Germany). The electrical conductivity of the samples was measured by a standard four-point probe resistivity measurement system (Keithley 2000 (Keithley Instruments Inc., Cleveland, OH, USA). Electrochemical measurements The electrochemical measurements were conducted using CR2026 coin cells with pure Li foil as the counter and reference electrode at room temperature. The working electrode consists of a test material (for example, EFG–S or rGO–S nanocomposite), carbon black (Super-P-Li) and polyvinylidene difluoride in a weight ratio of 7:2:1. The electrolyte used is 1.0 M Li bistrifluoromethanesulphonylimide in 1, 3-dioxolaneand 1, 2-dimethoxyethane (1:1 by volume) with 1.0 wt.% LiNO 3 additive. Cell assembly was carried out in an Ar-filled glovebox with the concentration of moisture and oxygen below 1.0 p.p.m. The galvanostatic charge/discharge tests were performed using a LAND CT2001A electrochemical workstation at different current densities within a cutoff voltage window of 1.5–3.0 V. The specific capacity is calculated based on the mass of sulphur. CV study was conducted using a CHI 660A electrochemical workstation between 1.5 and 3.0 V at a scan rate of 0.1 mV s −1 . Electrochemical impedance spectroscopy was performed using a CHI 660D electrochemistry workstation by applying an ac amplitude of 5 mV over the frequency range from 0.01 to 10 5 Hz. Computational method All calculations have been performed at the B3LYP/6-31g+(d) level of DFT using Gaussian 09 package. A large polyaromatic hydrocarbon molecule consisting of 24 C atoms and 12 H atoms was constructed to represent the graphene. The binding energy ( E ) is defined as the energy difference between EFG system with Li 2 S adsorbed ( E total ) and the summation of Li 2 S molecule ( E 1 ) and EFG system ( E 2 ): E = E 1 + E 2 − E total . Basis set superposition error has been considered in the calculation of binding energy. How to cite this article: Wang, Z. et al. Enhancing lithium–sulphur battery performance by strongly binding the discharge products on amino-functionalized reduced graphene oxide. Nat. Commun. 5:5002 doi: 10.1038/ncomms6002 (2014).